Super switching and control of in-plane ferroelectric nanodomains in strained thin films With shrinking device sizes, controlling domain formation in nanoferroelectrics becomes crucial. Periodic nanodomains that self-organize into so-called ‘superdomains’ have been recently observed, mainly at crystal edges or in laterally confined nanoobjects. Here we show that in extended, strain-engineered thin films, superdomains with purely in-plane polarization form to mimic the single-domain ground state, a new insight that allows a priori design of these hierarchical domain architectures. Importantly, superdomains behave like strain-neutral entities whose resultant polarization can be reversibly switched by 90°, offering promising perspectives for novel device geometries. Understanding and controlling domain formation in ferroelectrics at the nanoscale is interesting from a fundamental point of view and also of great technological importance. Increasing miniaturization in ferroelectric materials allows creating complex domain structures, offering novel functionalities [1] , [2] , [3] , [4] that could be particularly useful for the development of nanoelectronic devices. Most studies in thin films focus on domain patterns with up/down polarization for ferroelectric memories, while domain structures with purely in-plane polarization have not been much investigated. However, such structures are potentially useful, for example, in optical devices where in-plane domains, with vertical domain walls, could be manipulated optically, or in ultra-thin films, where avoiding depolarization field effects is necessary. Within the past decade, complex domain patterns (such as flux-closures and vortices) have been predicted to form in ferroelectrics as their dimensions are reduced [5] , [6] , [7] , [8] , [9] , [10] , [11] , motivating experimental work aimed to reveal such complex topological arrangements of electrical dipoles. Within the last 5 years, several experimental studies have been focused on the effect of geometrical confinement on novel nanoscale domain patterns [3] , [4] , especially in lamellae and small-scale dots from bulk single crystals of BaTiO 3 (refs 12 , 13 , 14 , 15 , 16 ), PbZr (1− x ) Ti x O 3 (PZT) [17] and Pb(Zn 1/3 Nb 2/3 ) (1− x ) Ti x O 3 (PZN-PT) [18] . A few studies were also conducted on disk-shaped thin film capacitor structures of PZT [19] , [20] . Exotic dipole arrangements have been evidenced but their formation remains not fully understood. Recently, complex domain structures have also been observed to occur spontaneously at grain boundaries (in PZT films) [21] , and heterointerfaces in thin ferroelectric films (of PZT and BiFeO 3 ) [22] , [23] . First results on their control by applying external electric fields (in PZT [21] and BiFeO 3 (ref. 1 )) appear very promising for the development of new nanoelectronic devices. It is, therefore, essential to understand the effect of geometry, electrical boundary conditions and local strains on the domain architectures in ferroelectrics. In ferroelectric thin films, epitaxial strain can be used as an additional degree of freedom to tune the domain configuration. Intensive theoretical work has thus been conducted on several ferroelectric materials in order to predict the changes of ferroelectric domain structures induced by strain [24] , [25] , [26] , [27] , [28] , [29] . Experimentally, epitaxial strain is typically created by growing high-quality thin films on suitable substrates [30] . A perfect control of the epitaxy is crucial in order to ensure domain formation as the only mechanism to relieve misfit stresses. However, the limited number of available substrates prevents continuous tuning of the epitaxial strain in one given material. In order to control the magnitude of the epitaxial strain in a continuous manner, from compressive to tensile, and access the whole diversity of available phases, a suitable combination of composition and substrate can be used. The substitution of Pb by Sr in Pb x Sr 1− x TiO 3 (PST) thin films grown epitaxially on (110)-DyScO 3 induces an increased tensile strain, predicted to stabilize a ferroelectric domain structure with purely in-plane polarization [31] , [32] . In this work, we use epitaxial growth and strain in extended PST thin films to stabilize and control a complex multiscale domain pattern with a purely in-plane polarization, which can be easily switched by 90° by a scanning probe. We show that 90° a 1 -a 2 stripe domains self-organize in distinct bundles, or superdomains, at larger scales, and we propose that this happens as a result of the competition between the preferred polar direction of the polydomain and the single-domain ground states. Unlike previous reports in laterally confined objects, where significant depolarizing fields are expected to affect the domain formation, our results prove that these hierarchical domain arrangements, forming flux-closure states, can be stabilized in extended thin films, where strain-equivalent superdomains are created to emulate the single-domain ground state. Importantly, despite the inherent difficulty to switch in-plane polarizations, the hierarchical domain organization allows the polarization in these films to be manipulated from the top surface, with the in-plane electric field available through a scanning probe [1] . The control of such domain architecture at two scales offers promising perspectives to design novel electronic devices based on thin films with vertical domain walls (DWs) and no effect of depolarizing field. Strain state and structure of Pb x Sr 1− x TiO 3 thin films In pure PbTiO 3 thin films grown on (110)-DyScO 3 , a tensile strain of 1.1% induces a usual a-c domain structure with periodic ferroelastic domains of alternating in-plane ( a domain) and out-of-plane ( c domain) ferroelectric polarization, as simply sketched in Fig. 1c (refs 33 , 34 , 35 ). In fact, the differences in a and c lattice parameters induce a non-flat surface with a twinned roof-like structure that makes this domain architecture directly observable in the film topographic image ( Fig. 1a ) [35] . X-ray diffraction (XRD) reciprocal space mapping (RSM) shows the presence of a and c domains, as well as additional intensity oscillations in the diffuse scattering because of their periodic arrangement [33] , [34] , [35] . In Pb x Sr 1− x TiO 3 films, by substituting Pb by Sr (decreasing x ), the tensile strain can be continuously increased. Both in-plane and out-of-plane lattice parameters have been measured by XRD to precisely characterize the films strain state as a function of composition. As expected, the strain state is found to be strongly dependent on the Pb content ( x ): the higher the x , the larger the unit cells tetragonality and the more difficult to keep the strain when increasing the thickness. Consequently, although 6-nm-thick films maintain the strain in the whole composition range under investigation ( x =0.55–1), 12- and 30-nm-thick films are only fully strained for x ≤0.7 and x ≤0.65, respectively. Lowering the Pb content to x =0.55, the films can remain fully strained up to a thickness of 100 nm or more. 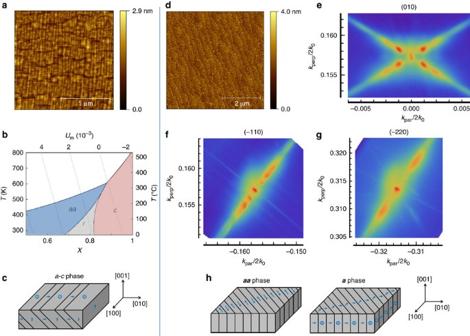Figure 1: Topography and ferroelectric phases of PbxSr1−xTiO3thin films. (a) AFM image (2 × 2 μm2) of a PbTiO3(50 nm) film, with ana-cdomain structure as sketched inc. (b) Phase diagram versus composition for PbxSr1−xTiO3(PST) strained on DyScO3as calculated using the Landau-Devonshire theory (the misfit strainUmis defined with respect to the lattice parameters of the extrapolated PST cubic phase)31. AFM image (5 × 5 μm2) (d) and in-plane reciprocal space maps (e–g) around the (010), (−110) and (−220) reflections, respectively, of a completely strained 30-nm-thick PST thin film (x=0.65). The axes are in units of 2k0, wherek0=2π/λwithλ=1.2398 Å. (h) Schematic view of the two possible ferroelectric structures:aaphase with 180° domain walls (left) andaphase with 90° domain walls (right). Figure 1: Topography and ferroelectric phases of Pb x Sr 1−x TiO 3 thin films. ( a ) AFM image (2 × 2 μm 2 ) of a PbTiO 3 (50 nm) film, with an a-c domain structure as sketched in c . ( b ) Phase diagram versus composition for Pb x Sr 1− x TiO 3 (PST) strained on DyScO 3 as calculated using the Landau-Devonshire theory (the misfit strain U m is defined with respect to the lattice parameters of the extrapolated PST cubic phase) [31] . AFM image (5 × 5 μm 2 ) ( d ) and in-plane reciprocal space maps ( e – g ) around the (010), (−110) and (−220) reflections, respectively, of a completely strained 30-nm-thick PST thin film ( x =0.65). The axes are in units of 2 k 0 , where k 0 =2 π / λ with λ =1.2398 Å. ( h ) Schematic view of the two possible ferroelectric structures: aa phase with 180° domain walls (left) and a phase with 90° domain walls (right). Full size image First, we take a look at films of 30 nm in thickness with x ≤0.65, which are fully strained, that is, they present the same in-plane lattice parameter as the DyScO 3 substrate. Orthorhombic (110)-DyScO 3 substrates do not have a totally squared in-plane lattice, however, the difference between the two in-plane parameters is small: the two in-plane lattice directions are [1–10] and [001], which we shall name a -axis and b -axis, respectively, corresponding to pseudo-cubic lattice parameter of 3.943 and 3.945 Å (ref. 36 ). Along these axes lie the [100] and [010] in-plane lattice directions of the PST films. The films out-of-plane lattice parameter being smaller than the in-plane value indicate an in-plane orientation of the polarization in this composition range [31] , [32] . This is consistent with a transition to an in-plane ferroelectric phase predicted under increasing tensile strain (blue area in Fig. 1b ) [31] . The transition to the in-plane phase takes place at different compositions for different thicknesses (at x =0.7 for 6-nm-thick films and at x =0.65 for 12- and 30-nm-thick films). In this in-plane polarized phase, the domain structure cannot be evidenced from the films topography, as expected. The atomic force microscopy (AFM) images show steps of one unit cell height ( Fig. 1d ), reflecting the substrate’s terraces and the high quality of the epitaxial growth. The lack of out-of-plane polarization is confirmed by piezoforce microscopy (PFM) measurements, as it will be discussed later. The domain structure in the in-plane-oriented ferroelectric phase has been studied from synchrotron XRD RSMs around various reciprocal lattice points. Such maps are presented in Fig. 1e–g for a 30-nm-thick PST film ( x =0.65). These XRD data are consistent with any in-plane ferroelectric periodic domain structure with DWs perpendicular to the in-plane <110> directions (see Supplementary Note 1 ). The two possible uncharged domain structures with these types of walls are presented in Fig. 1h : the aa phase with anti-parallel polarization 180° domains and the a phase with head-to-tail polarization (also called a 1 - a 2 or 90° domains) [25] . Periodic in-plane domain architecture at two length scales In-plane PFM has been performed in order to determine with certainty the ferroelectric domain structure in the in-plane polarized phase. The study of a fully strained 30-nm-thick PST film with x =0.65 is presented in Fig. 2 . First, very well-defined periodic domains with in-plane polarization are observed, with a periodicity along the <110> directions and a domain period of 46 nm, in good agreement with the XRD results. No response has been observed while measuring the vertical PFM signal (except the usual contrast attributed to the cantilever buckling effect in the presence of in-plane polarization) [14] , confirming the absence of an out-of-plane component of polarization. 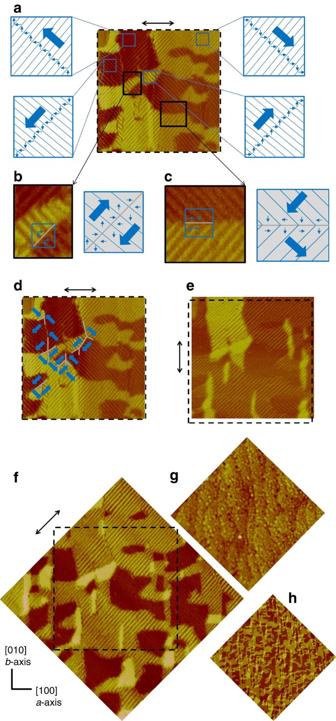Figure 2: Ferroelectric-ferroelastic domain architecture by in-plane PFM. AFM and PFM pictures of an in-plane polarized 30-nm-thick PST film withx=0.65. (a,d,e,f,h) Lateral PFM phase images (scale bar range, 0–70°) of areas of 2 × 2μm2(a,d,e), 2.8 × 2.8 μm2(f) and 10 × 10 μm2(h), measured by rotating the film by 0° (a,d), 90° (e) and 45° (f,h) with respect to the [100] axis. The direction of sensitivity to the polarization is indicated as double black arrows. The square area under investigation is visible in all scans and is marked surrounded by a dashed line. (g) Topographic picture corresponding to the PFM phase picture (f) (scale bar range, 0–4 nm). From these images, four types of areas are observed (marked by the blue squares ona), defining coarse-scale ‘superdomains’. The polarization orientation in the nanodomains is directed along thea- andb-axis, in agreement with theaphase, and is represented by blue arrows for the four types of 90° rotated variant. The boundary between two ‘superdomains’ can be 180° (enlarged imageb) or 90° domain walls (DWs; enlarged imagec). Wide blue arrows onddemonstrate the net polarization within the ‘superdomains’, with an example of 180° DWs, 90° DWs and a more complex flux-closure pattern. Figure 2: Ferroelectric-ferroelastic domain architecture by in-plane PFM. AFM and PFM pictures of an in-plane polarized 30-nm-thick PST film with x =0.65. ( a , d , e , f , h ) Lateral PFM phase images (scale bar range, 0–70°) of areas of 2 × 2μm 2 ( a , d , e ), 2.8 × 2.8 μm 2 ( f ) and 10 × 10 μm 2 ( h ), measured by rotating the film by 0° ( a , d ), 90° ( e ) and 45° ( f , h ) with respect to the [100] axis. The direction of sensitivity to the polarization is indicated as double black arrows. The square area under investigation is visible in all scans and is marked surrounded by a dashed line. ( g ) Topographic picture corresponding to the PFM phase picture ( f ) (scale bar range, 0–4 nm). From these images, four types of areas are observed (marked by the blue squares on a ), defining coarse-scale ‘superdomains’. The polarization orientation in the nanodomains is directed along the a - and b -axis, in agreement with the a phase, and is represented by blue arrows for the four types of 90° rotated variant. The boundary between two ‘superdomains’ can be 180° (enlarged image b ) or 90° domain walls (DWs; enlarged image c ). Wide blue arrows on d demonstrate the net polarization within the ‘superdomains’, with an example of 180° DWs, 90° DWs and a more complex flux-closure pattern. Full size image A careful study of the change of contrast by rotating the film proves that the in-plane polarization phase is the a phase presented in Fig. 1h with favourable head-to-tail polarization (uncharged DWs; see Supplementary Note 2 ). As observed in Fig. 1b , the Landau Devonshire approach predicted an aa phase in that region of the phase diagram [31] . This is the same ground state as found for pure PbTiO 3 under tensile strain [25] , [28] . However, in both cases, domain formation was neglected. Taking domain formation into account, calculations have shown the stabilization of the a phase, instead of the aa phase, for the region of the phase diagram with purely in-plane polarization [29] , which is in agreement with our experimental results. In the a phase, the domains are not only ferroelectric but also ferroelastic, unlike in the aa phase. Although domain formation would not be expected in the aa phase, in the a phase it can be easily understood as an efficient way to minimize the elastic energy (see Supplementary Note 3 ) [37] . These small scale nanodomains are seen to be arranged in four types of areas, related by 90° rotations, as observed on the lateral PFM pictures (marked by the blue squares in Fig. 2a ). These variants define micron-size ‘superdomains’ with a resultant in-plane component of polarization along the [110] and [1–10] directions (see wide blue arrows). Similar patterns have been observed in single crystals of BaTiO 3 (lamellae and dots) [12] , [14] , [15] , dots of PZT [17] and lamellae of PZN-PT [18] , as well as in relatively thick PZT and PbTiO 3 films [38] , [39] , which included a fraction of domains with out-of-plane polarization and partial strain relaxation by dislocations. The DWs between superdomains are observed along both <100> and <110> crystallographic directions (see Fig. 2h ). We have found 90°-type superdomain walls ( Fig. 2c ), if the periodicity direction rotates by 90°, and 180°-type superdomain walls ( Fig. 2b ) with no change of periodicity direction. The latter type appears to be less abundant in the PST thin films. Within the PFM resolution, these two types of DWs between superdomains seem to be locally charged. However, McGilly et al . [14] have recently investigated such type of apparently charged 180° DWs in BaTiO 3 by transmission electron microscopy and they evidenced zigzag bundle boundaries composed of local 180° DWs, forming continuous chains of adjacent flux closure and quadrupole states. It is likely that we have similar structures in our PST films, which would then form charge-neutral 180° superdomain boundaries. In some areas of the PST films, the four superdomain variants are present and arranged in 90° DWs to create flux-closure patterns at larger scales, in which the resultant in-plane polarization step-rotates from one quadrant to the next ( Fig. 2d ). Different quadrant arrangements can be observed, such as a fourfold vertex and several threefold wall junctions that are connected to each other by 180° DWs. Four 90° domain boundaries that intersect at a single point will create energetically unfavourable core singularities and rarely were observed in our PST films. Instead, flux closure objects are split into two threefold junction points connected by a 180° superdomain boundary, as discussed in ref. 18 . Complex domain patterns with flux closure objects at two different length scales have only been reported in ferroelectrics recently and their physical origin has remained unclear [18] . In dots of single crystals, significant in-plane depolarizing fields can be present, because of the reduced objects lateral size, and induce flux closure loops. Such strong effect of lateral depolarizing fields has been reported by McGilly et al . in BaTiO 3 single crystals dots [13] , [15] . A favourable formation of quadrants facilitating flux-closure at the mesoscale has been observed in vacuum [13] , whereas 180° superdomains have been evidenced in air [15] , showing the effect of surface charges and depolarizing fields on the domains architecture. The present work shows that strong lateral depolarizing fields are not needed in order to create hierarchical domain structures with flux-closure objects on continuous films. According to the predictions, although 90° stripe a 1 -a 2 nanodomains are the ground state of the polydomain strained film [29] , a hypothetical single-domain strained film would show an aa phase with polarization along the in-plane pseudocubic <110> directions [31] . The formation of superdomains mimics such single-domain ground state by creating strain-equivalent regions with average polarization oriented along the <110> directions. Thickness dependence of domain structure In the in-plane ferroelectric phase (composition range x =0.55–0.7) [31] , the domain size (or domain periodicity) does not appear to change much with the Pb content, most likely because of the relatively small changes in the magnitude of the strain in this composition range. However, the domain periodicity is strongly affected by the film thickness. The well-defined periodicity of the nanodomains increases with the film thickness, as it is well known for ferroelastic domains. The RSMs around the (−110) Bragg peak of PST films with x =0.55, in Fig. 3 , show that the satellite spacing decreases when increasing thickness. The evolution of the in-plane a domain period ( w ) with the thickness ( d ) for completely strained films is presented in Fig. 3d . It is worth noticing that for this composition a film thickness higher than 6 nm is required to develop enough strain and induce domain formation. The measured domain period as a function of film thickness is consistent with Roytburd’s square root law for ferroelastic domains [40] , [41] , as also observed in 90° a-a domains in BaTiO 3 lamellae [12] . For fitting the experimental data to Roytburd’s model, we use the lattice parameters of the film and the substrate (and thus the strain values) at room temperature, as the domain freezing temperature is not known at this point. The experimental data of our PST-strained films are well fit using a DW formation energy density of 26 mJ m − 2 . This value for a-a 90° DWs in strained films is of the same order as those estimated by Stemmer et al . [42] for a-c 90° DWs (that is, walls between in-plane and out-of-plane polarized domains) in relaxed PbTiO 3 films and those calculated by Meyer and Vanderbilt [43] using first-principles calculations for a-c 90° domains in relaxed PbTiO 3 films (at 0 K and excluding substrate clamping). 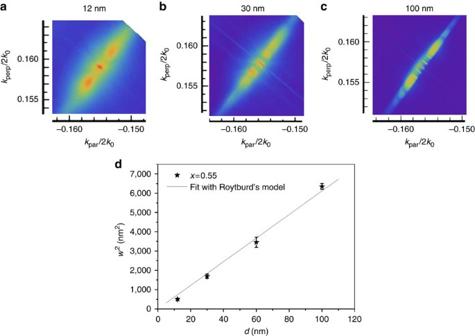Figure 3: Evolution of domain size. X-ray in-plane reciprocal space maps around the (−110) reflection of completely strained PST thin films forx=0.55 at different thickness (a)d=12 nm, (b)d=30 nm and (c)d=100 nm. Axes are in units of 2k0, wherek0=2π/λwithλ=1.2398 Å. The intensities scales (colour differences) are in logarithm scale. (d) Domain period (w) of the nanodomains as a function of the films’ thickness (d) in theaphase. The solid line is the linear fit, in agreement with Roytburd’s law40,41. Figure 3: Evolution of domain size. X-ray in-plane reciprocal space maps around the (−110) reflection of completely strained PST thin films for x =0.55 at different thickness ( a ) d =12 nm, ( b ) d =30 nm and ( c ) d =100 nm. Axes are in units of 2 k 0 , where k 0 =2π/ λ with λ =1.2398 Å. The intensities scales (colour differences) are in logarithm scale. ( d ) Domain period ( w ) of the nanodomains as a function of the films’ thickness ( d ) in the a phase. The solid line is the linear fit, in agreement with Roytburd’s law [40] , [41] . Full size image We also observe that one of the four superdomain variants becomes more favourable when the film thickness increases ( Fig. 4 ), leading to very long anisotropic periodic nanodomains with a most favourable resultant polarization along one of the four in-plane <110> diagonals. This is clearly seen in PST films at x =0.55 that can stay fully strained up to thicknesses of 100 nm. As the film thickness increases, the elastic energy associated to the formation of walls between the superdomain variants increases, so that it becomes energetically more favourable to present only one type of variant [44] . 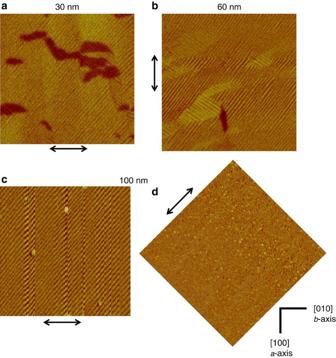Figure 4: Effect of film thickness on domain structure. Lateral PFM phase images on PST films withx=0.55 (at the in-plane polarizeda-phase) and thicknesses of 30 nm (a, picture size 2 μm), 60 nm (b, picture size 3 μm) and 100 nm (c, picture size 3 μm). The latter sample shows completely parallel domain walls for areas as large as 10 μm (d, picture size 10 μm). Colour scale range=0–70°. Figure 4: Effect of film thickness on domain structure. Lateral PFM phase images on PST films with x =0.55 (at the in-plane polarized a -phase) and thicknesses of 30 nm ( a , picture size 2 μm), 60 nm ( b , picture size 3 μm) and 100 nm ( c , picture size 3 μm). The latter sample shows completely parallel domain walls for areas as large as 10 μm ( d , picture size 10 μm). Colour scale range=0–70°. Full size image Switching of in-plane polarization Interestingly, we have been able to switch the polarization in a phase PST films. An in-plane electric field is available in the standard out-of-plane geometry, that is, by applying a bias between the bottom electrode and a metallic AFM tip, as reported by Blake et al . [1] Fig. 5a shows the as-grown domain structure in an a phase 30-nm-thick PST film ( x =0.65). The switching of the in-plane polarization in nanodomains is associated to a rotation by 90° of the DWs (and, thus, to a switching by 90° of the resultant in-plane polarization) in the superdomains (marked by big blue arrows on Fig. 5b,c ). The in-plane switching mechanism is described in more detail in the next paragraph. 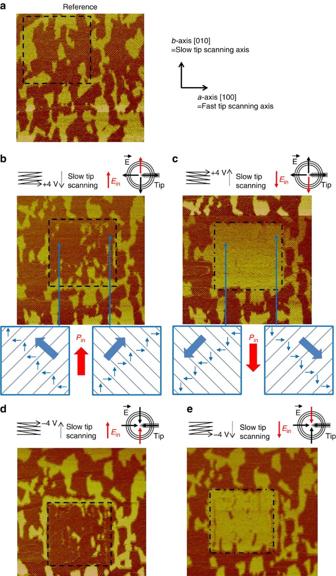Figure 5: Control of the in-plane polarization switching (30-nm-thick PST film,x=0.65). PFM phase pictures (scale bar, 70–100°) of the as-grown state (a) and after applying a bias of 4 V (b,c) and −4 V (d,e) to the AFM tip in the area delimited by the dashed square during scanning in the b− direction (b,e) or b+ direction (b,c). The tip orientation and the in-plane electric fields, causing the switching along the slow scanning axis, are presented in sketches (same manner as in Balke’s article1). Figure 5: Control of the in-plane polarization switching (30-nm-thick PST film, x =0.65). PFM phase pictures (scale bar, 70–100°) of the as-grown state ( a ) and after applying a bias of 4 V ( b , c ) and −4 V ( d , e ) to the AFM tip in the area delimited by the dashed square during scanning in the b− direction ( b , e ) or b+ direction ( b , c ). The tip orientation and the in-plane electric fields, causing the switching along the slow scanning axis, are presented in sketches (same manner as in Balke’s article [1] ). Full size image All PFM pictures on Fig. 5 have been obtained by a fast (slow) tip scanning along the a -axis ( b -axis). During the switching, the bias has been applied to the tip while scanning the sample in the b+ direction (from bottom to top of the picture) or in the b− direction (from top to bottom of the picture). In the as-grown state, the four types of superdomain variants can be observed, as previously discussed. After applying a tip bias (positive or negative), a preferred stabilization of the two variants with the same polarization along the b -axis (slow scanning axis) is clearly obtained (see Fig. 5b,c ). Applying a positive tip bias while scanning in the b− direction ( Fig. 5b , dark colour) or applying a negative tip bias while scanning in the b+ direction ( Fig. 5d ), allows stabilizing the same set of variants. A positive tip bias with a scanning in the b+ direction ( Fig. 5c ) has also the same effect as a negative tip bias with a scanning in the b− direction ( Fig. 5e ): a preferred stabilization of the two variants with the polarization parallel to the in-plane applied field. These data strongly suggest that the in-plane component of the applied field under the tip certainly has a role in the switching mechanism of the in-plane polarization, as also demonstrated by Balke et al . [1] in BiFeO 3 thin films. A detailed description of the effect of the in-plane electric fields is presented in the Supplementary Note 4 . Looking at the data, though, the mechanism of in-plane switching seems more complex, with an associated 90° rotation of the DWs. Simply switching by 180°, the in-plane polarization in the nanodomains along the slow scanning axis (vertical in the figures) would induce charged DWs between nanodomains. Although charged DWs can exist under certain conditions [45] , it is often not the most favourable configuration and, indeed, Fig. 5 shows that head-to-head and tail-to-tail domain configurations are avoided in this case. Thus, what the experiments are revealing is that the in-plane electric field induces, next to the 180° switching of some particular areas, the 90° rotation of the polarization on the adjacent areas, changing the orientation of the domains walls and avoiding head-to-head and tail-to-tail configurations. This seems to be a very efficient mechanism by which four ninths of the sample can remain unswitched, nevertheless producing a net total moment in the desired direction (see Supplementary Fig. 1 ). As discussed previously in this article, the structure of PST films is close to cubic, with a relatively small a/c ratio, which most likely enables the 90° rotation. Modelling polarization dynamics would help better understand the switching mechanism of purely in-plane polarization under the PFM tip. Such study would require a precise determination of the electric field components under the tip, but is beyond the purpose of this work. Even if the exact mechanism of in-plane polarization switching remains to be theoretically proven, our results clearly demonstrate that it is possible to switch a purely in-plane polarized thin film using PFM. The reason why this is possible is the self-arrangement of the nanodomains in superdomains with space-averaged polarization pointing along the diagonals of the pseudocubic lattice. It is the presence of superdomains that allows switching of the purely in-plane polarization because, unlike the nanodomains, the different superdomain variants are strain-equivalent and they are therefore not elastically pinned to neighbouring superdomains. This type of switching mechanism is favoured by the small tetragonality of the samples and the very small barrier for the motion of 90° DWs [43] . Because we have shown that superdomains are formed also in regular extended samples with competing (single-domain versus poly-domain) ground states, this work paves the way towards a more deterministic ‘writing’ of in-plane domain structures in ferroelectric films. To conclude, we show that with sufficient control of the epitaxial growth and strain in extended thin films, it is possible to stabilize and control complex domain architectures at two different scales, yielding periodic ferroelectric nanodomains with purely in-plane polarization and organized in strain-equivalent superdomains, so far mainly observed in laterally confined samples. Such multiscale domain arrangement emerges from the differences in the ground state of the poly-domain and single-domain strained films (superdomains emulate the single-domain ground sate) and it facilitates domain switching. In this way, a pure in-plane polarization can be switched from the top surface with the in-plane electric field created by a scanning probe. Epitaxial growth Pb-rich PST thin films with x =0.55–1 (of 6, 12, 30, 60 and 100 nm thickness) were grown on (110)-oriented DyScO 3 substrates (from CrysTec GmbH) by pulsed laser deposition using a pulsed KrF excimer laser ( λ =248 nm), from Pb x Sr 1−x TiO 3 targets with 4 atomic % excess lead. The substrates were treated to get a single ScO 2 termination [33] , [46] , allowing the growth of high-quality SrRuO 3 bottom electrodes. The growth was followed in situ by reflection high-energy electron diffraction and the films thickness was determined from the reflection high-energy electron diffraction intensity oscillations, together with X-ray reflectivity. The thickness of the SrRuO 3 layer was 8 nm in order to get fully strained films and thus keep the lattice parameters of the substrate for the deposition of PST. The growth parameters were tuned to optimize the epitaxial quality of PST films (temperature of 580 °C, oxygen partial pressure of 0.06 mbar, 2 J cm − 2 laser fluence, laser frequency of 10 Hz, spot size of 0.8 mm 2 and a target-substrate distance of 50 mm). X-ray diffraction The epitaxial structure and strain state of the films were studied by XRD in both normal and grazing incidence geometry. We used the facilities of both the HASYLAB P08 beamline (Petra III-DESY, Desy), for grazing incidence measurements, and a Panalytical X'Pert MRD Cradle (four axes) laboratory diffractometer. The wavelengths used were 1.2398 and 1.5406 Å, respectively. Atomic force and piezoresponse force microscopies The films were characterized using AFM in tapping mode, to access the morphology, and using PFM (both in-plane and out-of-plane modes) to study the ferroelectric domain structure and switching. For PFM measurements, our Dimension V (Veeco/Bruker) microscope was equipped with conductive Co/Cr-coated silicon tips (spring constant 5 N m −1 ) and an alternating voltage was applied between the tip and the SrRuO 3 bottom electrode at a frequency of about 25 kHz for domain mapping, with a voltage amplitude in the 0–5 V range. How to cite this article: Matzen, S. et al . Super switching and control of in-plane ferroelectric nanodomains in strained thin films. Nat. Commun. 5:4415 doi: 10.1038/ncomms5415 (2014).